BMI1–RING1B is an autoinhibited RING E3 ubiquitin ligase Polycomb repressive complex 1 (PRC1) is required for ubiquitination of histone H2A lysine 119, an epigenetic mark associated with repression of genes important in developmental regulation. The E3 ligase activity of PRC1 resides in the RING1A/B subunit when paired with one of six PCGF partners. The best known of these is the oncogene BMI1/PCGF4. We find that canonical PRC1 E3 ligases such as PCGF4–RING1B have intrinsically very low enzymatic activity compared with non-canonical PRC1 RING dimers. The structure of a high-activity variant in complex with E2 (PCGF5–RING1B–UbcH5c) reveals only subtle differences from an earlier PCGF4 complex structure. However, two charged residues present in the modelled interface with E2-conjugated ubiquitin prove critical: in BMI1/PCGF4, these residues form a salt bridge that may limit efficient ubiquitin transfer. The intrinsically low activity of the PCGF4–RING1B heterodimer is offset by a relatively favourable interaction with nucleosome substrates, resulting in an efficient site-specific monoubiquitination. Polycomb group (PcG) proteins are critical regulators of Hox gene expression during development, originally discovered through genetic screens in Drosophila [1] . The PcG proteins segregate into two major polycomb repressive complexes, PRC1 and PRC2 (refs 2 , 3 , 4 ). Each of these PRCs carries a primary enzymatic function important in epigenetic gene silencing: PRC2 is the Histone H3K27 methyl transferase, while PRC1 is an E3 ubiquitin (Ub) ligase that transfers the mono-Ub mark to the C-terminal tail of Histone H2A at K118/K119. Canonical PRC1 E3 ligase activity is conferred by a RING-class [5] , [6] heterodimer, BMI1 (PCGF4) or MEL-18 (PCGF2) paired with RING1A/B [7] , [8] , [9] . PRC1 is also capable of chromatin compaction, a function not requiring histone tails, and this activity appears important in gene silencing [10] . Histone H2A K119ub is a modification that is readily detected in bulk chromatin, and it has been estimated that, depending on cell type and study, ∼ 1% to over 10% of total cellular H2A may carry this mark. The importance of H2A K119ub in PRC1-enforced gene repression has been studied in several systems [11] , [12] , [13] (reviewed in refs 14 , 15 ). Introduction of a catalytically inactive RING1B mutant into Ring1A −/− Ring1B conditional knockout embryonic stem (ES) cells [12] established that H2A ubiquitination is dispensable for chromatin compaction but essential for maintaining repression of target genes and for maintaining ES cells in a dedifferentiated state. Although some details of PRC1 function are different in Drosophila [15] , it appears that H2A ubiquitination is again critical for a subset of PRC1 function [13] . In accord with the importance of H2A ubiquitination, the process is highly regulated: a number of H2A K119 deubiquitinases have been identified and assigned critical functions (recently reviewed in ref. 16 ). Human PRC1 subunits each have multiple paralogues, resulting in a large number of potential combinations [17] . In particular, the subunits necessary for E3 ligase activity, PCGF and RING1, are families of six and two paralogues, respectively ( Fig. 1 ; Supplementary Fig. 1 ). Recently, it has been appreciated through work in many labs that, in addition to canonical PRC1, several variant PRC1 complexes are present in mammalian cells [18] , [19] , [20] , [21] , [22] , [23] , [24] , [25] , [26] , [27] , [28] , [29] . These are defined by the PCGF family member present [23] , and the copurifying subunits also differ by complex subtype [22] , [23] , [25] . Opinions currently differ on which type of complex, canonical [25] or non-canonical [23] , [29] , may contribute more strongly to H2A K119 ubiquitination. However, very little data have been published comparing directly the two classes of ligases. 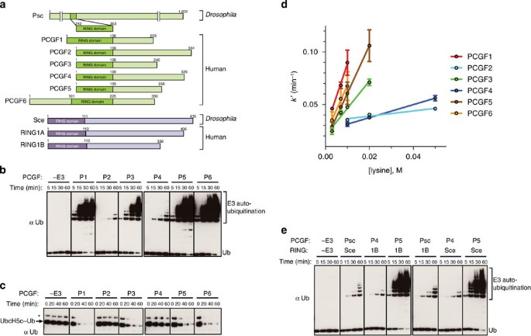Figure 1: E3 ligase activity of RING1B–PCGF complexes. Unless specified, RING1B is common to all E3 complexes, so only the identity of the PCGFs is shown (P1–P6). Reactions throughout were monitored by western blot (α-Ub) unless stated otherwise. (a) Human andDrosophilaPCGF (green) and RING1 proteins (purple). Boundaries of the RING domain constructs used in this study are shown. (b) Auto-ubiquitination by the various GST–RING1B–PCGF complexes. (c) Discharge of Ub from the UbcH5c∼Ub conjugate (‘∼’ represents a covalent thiolester bond) to excess solution lysine in the presence of the indicated E3 complex. The discharge assay is a direct readout of intrinsic E3 catalytic activity. * represents a band that appears to be UbcH5c conjugated to diUb (note discharge in parallel with E2∼Ub). (d) Rate of ubiquitin discharge from the indicated PCGF–RING1B–UbcH5c∼Ub complex. Reaction progress was monitored by discharge-induced fluorescence polarization (FP) changes of BODIPY-FL-labelled ubiquitin (see Methods andTable 1) and is plotted as apparent, pseudo first-order rate constant (k′app±s.d.) at the indicated lysine concentration. Rates were determined from duplicate measurements for PCGFs 1, 2 and 4. For PCGFs 3, 5 and 6, four replicates were averaged (except two replicates at 20 mM lysine). (e) Auto-ubiquitination by human,Drosophilaand human–Drosophilachimeric GST–RING1–PCGF complexes. Figure 1: E3 ligase activity of RING1B–PCGF complexes. Unless specified, RING1B is common to all E3 complexes, so only the identity of the PCGFs is shown (P1–P6). Reactions throughout were monitored by western blot (α-Ub) unless stated otherwise. ( a ) Human and Drosophila PCGF (green) and RING1 proteins (purple). Boundaries of the RING domain constructs used in this study are shown. ( b ) Auto-ubiquitination by the various GST–RING1B–PCGF complexes. ( c ) Discharge of Ub from the UbcH5c ∼ Ub conjugate (‘ ∼ ’ represents a covalent thiolester bond) to excess solution lysine in the presence of the indicated E3 complex. The discharge assay is a direct readout of intrinsic E3 catalytic activity. * represents a band that appears to be UbcH5c conjugated to diUb (note discharge in parallel with E2 ∼ Ub). ( d ) Rate of ubiquitin discharge from the indicated PCGF–RING1B–UbcH5c ∼ Ub complex. Reaction progress was monitored by discharge-induced fluorescence polarization (FP) changes of BODIPY-FL-labelled ubiquitin (see Methods and Table 1 ) and is plotted as apparent, pseudo first-order rate constant ( k ′ app ±s.d.) at the indicated lysine concentration. Rates were determined from duplicate measurements for PCGFs 1, 2 and 4. For PCGFs 3, 5 and 6, four replicates were averaged (except two replicates at 20 mM lysine). ( e ) Auto-ubiquitination by human, Drosophila and human– Drosophila chimeric GST–RING1–PCGF complexes. Full size image Here we examine enzymatic properties of all the six core RING–RING heterodimers, and we find unexpectedly a profound difference in intrinsic catalytic activity between canonical and non-canonical PCGF–RING1 E3s. Through structural and mutagenesis studies, we identify a novel and conserved mechanism through which canonical PCGF2/4 limits the activity of RING1. In addition, we demonstrate that, contrary to expectation [6] , [30] , PCGF–RING1 ligases use a mode of Ub recognition and activation [31] highly similar to that recently discovered for homodimeric RING E3s [30] , [32] , [33] and monomeric RINGs CBL-B and RNF38 [34] , [35] . In contrast to the differences in their intrinsic catalytic activities, we find all the six PCGF–RING1 heterodimers to be robust H2A ligases in an assay using purified components. Mutation of residues implicated in nucleosome recognition, and distinct from the ubiquitin interaction surface, reveals that canonical PCGF4–RING1B overcomes poor intrinsic catalytic activity by engaging in a highly complementary interaction with the nucleosome substrate. Canonical PRC1 E3 ligases have very low intrinsic activity PCGF4 (BMI1) and PCGF2 (MEL-18) form equivalent protein complexes (designated PRC1.4 and PRC1.2, respectively) that correspond most closely to canonical PRC1 (ref. 23 ). The other four PCGF proteins are present in three distinct protein complexes (PRC1.1, PRC1.3/1.5 and PRC1.6) that differ in targeting subunits, bind to different genomic loci, and regulate expression of different genes [23] . Nevertheless, these variant complexes all include RING1B, and, therefore, it might be presumed that they are active E3 ligases. Indeed, endogenous PRC1.1 (BCOR) [19] and PRC1.6 (E2F6/PRC1L4) [21] complexes have been shown to have H2A K119 ubiquitination activity. We co-expressed RING domains from RING1B and each of the six human PCGFs ( Fig. 1a ) and purified the minimal, core E3 complexes for comparison. To test sensitively for E3 activity, we first used an auto-ubiquitination assay in which a glutathione S-transferase (GST) tag on RING1B acts as a pseudo-substrate. Surprisingly, the canonical and non-canonical RING1B–PCGF complexes show very different levels of activity ( Fig. 1b ). The core complexes corresponding to canonical PRC1 (those including PCGF4 and PCGF2) show very low E3 ligase activity (PCGF low-activity group), whereas the core complexes of PCGFs 1, 3, 5 and 6 are strongly active in this assay (PCGF high-activity group). Because the GST pseudo-substrate could conceivably alter the behaviour of the complexes, we also removed the tag and evaluated the ability of the RING–RING complexes to catalyse discharge of E2 ∼ Ub to excess lysine (E2 discharge assay) [36] . As seen in the auto-ubiquitination assay, the PCGF complexes segregate into the two activity groups, with the PCGF high-activity group efficiently discharging Ub and the PCGF low-activity group showing only limited discharge of E2 ∼ Ub over the 60-min time course ( Fig. 1c ). To quantify differences in discharge rate over a range of lysine concentrations, we developed a fluorescence polarization (FP) assay. Fluorescent, tagged ubiquitin (exhibiting only modest FP signal because of its low molecular weight) was conjugated to E2 and driven to a higher polarization state by binding to excess E3. In the presence of lysine, a decrease in FP signal reflects reaction of lysine with E2 ∼ Ub ( Supplementary Fig. 2 ). Because discharge of E2 ∼ Ub to lysine typically requires a large excess of lysine over E2 ∼ Ub, the reaction is pseudo first-order with respect to E2 ∼ Ub concentration (with rate constants k ′). Second-order rate constants ( k 2 ) are obtained from the slope of k ′ versus lysine concentration ( Fig. 1d ). The results obtained are fully consistent with rate differences indicated from Fig. 1c . In particular, the four ‘high-activity’ ligases (RING1B heterodimers of PCGFs 1, 3, 5 and 6) are all of higher activity in the FP assay than are the PCGF low-activity variants. Comparison of the different PCGF–RING1B–E2 ∼ Ub reaction rates yielded k 2 values covering a range of ∼ 25-fold, with the nearest of the high- and low-activity PCGFs (PCGF3 and PCGF4, respectively) differing by more than fourfold in k 2 ( Table 1 ). Table 1 Apparent second-order rate constants ( k 2,app ) for discharge of activated ubiquitin to lysine from the indicated RING1B–PCGF–E2 ∼ Ub complex. Full size table The data above demonstrate large differences in activity for the PCGF–RING1B complexes. However, the PCGFs also heterodimerize with the very close RING1B relative, RING1A ( Supplementary Fig. 1b ). We wondered whether the activity profiles of the six RING1B–PCGF complexes might reflect different preferences for pairing with RING1 variants. The RING1A–PCGF complexes show the same activity differences as their RING1B–PCGF counterparts ( Supplementary Fig. 3a ), suggesting that these differences are dictated by the PCGF partner, not by the combination of a PCGF with the ‘preferred’ or ‘less-preferred’ RING1. Taken together, these data support a strong deficiency in the intrinsic catalytic competence of the canonical PRC1 complexes compared with other family members. The implication that the PCGF partner in the core complex regulates ligase activity is provocative in light of its previously understood role. The structure of PCGF4–RING1B–UbcH5c shows that the E2 binds to RING1B and that the PCGF4 RING domain does not physically contact E2 (ref. 37 ). In addition, a mutation on RING1B that impairs E2 recruitment (D56K on RING1B) rendered the RING1B–PCGF4 complex catalytically inactive, demonstrating that the PCGF4 RING domain lacks E3 ligase activity of its own [37] , [38] and suggesting instead that it acts to stabilize RING1B. One possible explanation for the robust activity of the PCGF high-activity complexes is that these RING domains can bind directly to E2 and thereby support E3 activity that supplements that of RING1B. We therefore prepared all the six PCGFs in complex with GST–RING1B(D56K). All complexes bearing the mutation in RING1B lacked activity ( Supplementary Fig. 3b ), demonstrating that none of the PCGFs is itself an active E3. Instead, it would appear that the PCGF strongly modulates activity of the core complex despite all contact with E2 occurring through the shared RING1B partner. One of the earliest members of the PCGF family to be characterized functionally is the D. melanogaster polycomb group (PcG) protein posterior sex combs (Psc; Fig. 1a ) [1] , [39] , [40] , [41] . Psc is the only PCGF protein present in Drosophila , and it pairs with the single RING1 orthologue sex combs extra (Sce, or dRING; Fig. 1a ) [42] , [43] . The function of the unique complex in Drosophila is similar to that of canonical human PRC1 (ref. 8 ). While the human and Drosophila RING1 orthologues show very high sequence identity, the PCGF orthologues do not ( Supplementary Fig. 1c,d ). We purified GST–Sce–Psc core RING–RING complex and found that it had only slightly higher auto-ubiquitination activity than its human counterpart (the PCGF4 complex; Fig. 1e ). To test more broadly the ability of the PCGF RING to regulate RING1 ligase activity, we made Drosophila –human chimeras with the RING1 component from one species in complex with the PCGF component from the other. Residues at the RING1–PCGF interface ( Supplementary Fig. 1a,b ) are highly conserved, and, accordingly, expression and purification of the chimeric complexes proved straightforward. The auto-ubiquitination activities of chimeric complexes correlated with the identity of the PCGF RING ( Fig. 1e ). In particular, Psc was capable of restraining the activity of human RING1B, while human PCGF5 could support a much higher level of activity from Sce than is seen with its natural partner Psc. This demonstrates that Sce is fully competent for robust E2 activation but also that it is kept in check by Psc. The finding that low intrinsic E3 ligase activity is enforced by both Psc and PCGF4, and is therefore preserved from Drosophila to human, suggests that it may be biologically important to closely regulate the catalytic rate of the canonical PRC1 complex. Structural features of the RING1B–PCGF5–UbcH5c complex Given that we find two activity classes of PCGF E3 ligases, we considered whether there might be a corresponding difference apparent in the structures of the E2–E3 complexes. 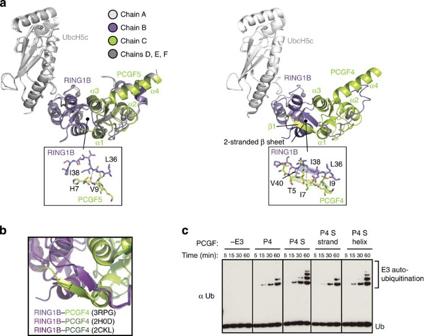Figure 2: Structural differences between PCGF5 and PCGF4 in complex with RING1B. (a) Overlay of the two complexes in the asymmetric unit in the crystal structure of RING1B–PCGF5–UbcH5c (chains A, B and C compared with chains D, E and F) is shown at left (root mean squared deviation 0.75 Å over 339 residues, using Coot SSM superpose67; the copy consisting of chains A, B and C is used in subsequent figures). The structure of the previously solved RING1B–PCGF4–UbcH5c (PDB code: 3RPG37) is shown at right for comparison. The PCGF4 and PCGF5 complexes are highly similar with an overall r.m.s.d of 1.11 Å over 340 residues. Helices within the PCGF are numbered α1 through α4. The β-strand labelled β1 on the PCGF4 cartoon is absent in PCGF5: insets show close-up views of the hydrogen-bonding pattern between RING1B and the PCGF5 or PCGF4 N termini. (b) Close-up view of the overlay of the two-stranded antiparallel β-sheet from previously solved RING1B–PCGF4 structures37,38,47. PDB codes are shown in parentheses. (c) Activity comparison of PCGF chimeric complexes exchanging strand β1 and/or helix α1 as monitored by western blot. All PCGFs are in complex with GST–RING1B. ‘P4 S’ (swap) denotes PCGF51–17PCGF418–109, ‘P4 S strand’ denotes PCGF51–8PCGF49–109and ‘P4 S helix’ denotes PCGF41–8PCGF59–17PCGF418–109. The crystal structure of PCGF5–RING1B–UbcH5c was determined to 2.00 Å by molecular replacement ( Table 2 ; Fig. 2a ). The structure of the RING–RING heterodimer within the ternary complex is closely similar to that found in the previously solved structure of RING1B–PCGF4–UbcH5c. Consistent with the mutagenesis studies above and the earlier structure (3RPG) [37] , the new structure shows RING1B bound directly to UbcH5c, with the PCGF partner making no contacts with the E2. The residues forming the interface between the PCGF and RING1B are highly conserved: of 18 interface residues, only two, both from helix α1, differ between PCGF4 and PCGF5 ( Supplementary Fig. 1a ). Furthermore, the structure of RING1B itself is highly similar in the two structures (root mean squared deviation of 0.69 Å over core residues 45–116 from 3RPG and chain B of the present structure) and, accordingly, few differences are seen in the structures of bound E2 or in the details of the UbcH5c–RING1B interface. In particular, the catalytically critical hydrogen bond [31] between RING1B R91 and the backbone carbonyl of UbcH5c Q92 is present in both the structures, consistent with an activated conformation of the E2. It is therefore not evident why one of the two E2s should be much more highly active in Ub transfer. Table 2 Data collection and refinement statistics. Full size table Figure 2: Structural differences between PCGF5 and PCGF4 in complex with RING1B. ( a ) Overlay of the two complexes in the asymmetric unit in the crystal structure of RING1B–PCGF5–UbcH5c (chains A, B and C compared with chains D, E and F) is shown at left (root mean squared deviation 0.75 Å over 339 residues, using Coot SSM superpose [67] ; the copy consisting of chains A, B and C is used in subsequent figures). The structure of the previously solved RING1B–PCGF4–UbcH5c (PDB code: 3RPG [37] ) is shown at right for comparison. The PCGF4 and PCGF5 complexes are highly similar with an overall r.m.s.d of 1.11 Å over 340 residues. Helices within the PCGF are numbered α1 through α4. The β-strand labelled β1 on the PCGF4 cartoon is absent in PCGF5: insets show close-up views of the hydrogen-bonding pattern between RING1B and the PCGF5 or PCGF4 N termini. ( b ) Close-up view of the overlay of the two-stranded antiparallel β-sheet from previously solved RING1B–PCGF4 structures [37] , [38] , [47] . PDB codes are shown in parentheses. ( c ) Activity comparison of PCGF chimeric complexes exchanging strand β1 and/or helix α1 as monitored by western blot. All PCGFs are in complex with GST–RING1B. ‘P4 S’ (swap) denotes PCGF5 1–17 PCGF4 18–109 , ‘P4 S strand’ denotes PCGF5 1–8 PCGF4 9–109 and ‘P4 S helix’ denotes PCGF4 1–8 PCGF5 9–17 PCGF4 18–109 . Full size image The primary differences between the PCGF4 and PCGF5 ternary complex structures are found at the N termini of the PCGF and RING1B. Electron density is absent for the first nine residues of RING1B in the PCGF5 complex (compared with the first 15 residues of RING1B in 3RPG), and it appears that this difference reflects a difference in crystal packing. For PCGF5, either the first four or first six residues are missing from the two copies in the asymmetric unit (compared with the first two residues for PCGF4 in 3RPG). The N terminus of PCGF4 (residues 5–9) forms a short two-stranded antiparallel β-sheet with residues 36–40 of RING1B ( Fig. 2a ), and this sheet is largely present in published structures of the E3 alone ( Fig. 2b ). In contrast, this structural element is not well formed in the PCGF5 complex. Two of five backbone hydrogen bonds present in the PCGF4 complex are present in one copy of PCGF5–RING1B ( Fig. 2a , insets); in the second copy, this entire element appears to be disordered. Sequence differences in strand regions of PCGFs 4 and 5 (‘TRIKI’ and ‘RKHLV’, respectively) reflect a difference in intrinsic β-sheet propensity, suggesting that the structural difference may exist in solution. The greater degree of structure in PCGF4 strand β1 and the sequence differences in the immediately following helix α1 (see above and Supplementary Fig. 1a ) suggested that this portion of the PCGF–RING1B interface might influence activation of UbcH5c. To test this, we replaced the first 17 residues of PCGF4 (the entire region that forms β1 and α1) with the corresponding segment from PCGF5; this resulted in a modest increase in E3 activity (P4 S; Fig. 2c ). Finer swaps of just β1 or just α1 revealed helix α1 to be the region associated with the observed increase in activity ( Fig. 2c ). Thus, it appears that the N-terminal regions of the PCGFs play some role in regulating Ub transfer from the E2 (presumably through propagation of a small structural difference through RING1B to the E2), but the effects do not nearly account for the large activity differences between the two classes of E3s. Ub conjugation does not enhance E2 affinity for PCGF E3s From the studies described above, we conclude that the RING1 ligases are strongly regulated by their PCGF partners, but it is not immediately evident how this is achieved. An interesting possibility is suggested by recent mechanistic work on RING E3s. It has been found that several RING–RING dimers have up to 60-fold greater affinity for E2 ∼ Ub than for E2 alone, with the additional affinity coming from interactions between Ub and the E3 (refs 30 , 32 ). This favourable interaction of E3 and Ub is thought to position Ub properly for transfer from E2 to substrate [30] , [31] , [32] . Interestingly, no such enhanced affinity for charged E2 binding to the RING1B–PCGF4 complex was observed [30] , but these authors did not characterize E2 interactions with other PCGF complexes. We asked whether the PCGF high-activity group complexes might exhibit enhanced affinity for E2 ∼ Ub. Because the E2 ∼ Ub thiolester bond is highly labile, we generated a stable isopeptide mimic of Ub-charged E2 from UbcH5c carrying the mutations C85K (to permit isopeptide bond formation) and S22R (to block an unwanted secondary interaction between Ub and UbcH5c [35] , [44] ). 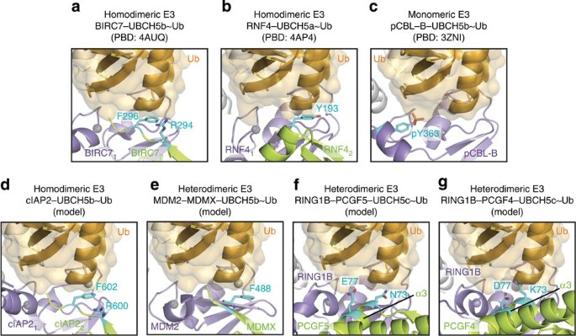Figure 3: Interactions between ubiquitin (Ub) and E3. (a–c) Close-up views of the E3-Ub interface from previously reported crystal structures. For the homodimeric E3s, Ub (orange) makes contacts with the E2-distal monomer (green). E3 residues shown in cyan mediate interactions with Ub. For the monomeric CBL-B, phosphorylation mediates the E3-Ub interaction. (d–g) Previous crystal structures were combined using structural overlays to generate models of E3–E2∼Ub complexes. A close-up view of the modelled E3-Ub interface is shown in each case (with RING monomers coloured as at top). Residues from the E3 that are expected to contact Ub are shown in cyan. (d) Model of cIAP2–UbcH5∼Ub complex. The experimental structure of cIAP2–UbcH5b (3EB6 (ref.45)) was overlaid with that of BIRC7–UbcH5b∼Ub (4AUQ30) by aligning the E2s. (e) Model of MDM2–MDMX–UbcH5∼Ub generated by aligning the MDM2 monomer from the MDM2–MDMX structure (2VJE70) with the E2 proximal BIRC7 monomer from 4AUQ30. (f,g) Models of PCGF5– and PCGF4–RING1B-UbcH5∼Ub generated by overlaying the structure reported here (f) or 3RPG (g) with 4AUQ30by aligning the E2s. The dissociation constant for E2 or E2 ∼ Ub binding to each immobilized E3 complex was determined using bio-layer interferometry (BLI; Table 3 , Supplementary Fig. 4 ). Comparing the PCGF complexes with one another, as well as binding of E2 to that of E2 ∼ Ub, we observe only very small differences in K D (no more than approximately twofold) and no trends that could explain the large differences in E3 ligase activity. Table 3 Dissociation constants ( K D ) for interactions between RING1B–PCGF complexes with either UbcH5c(S22R/C85K) ∼ Ub or UbcHc(S22R/C85K). Full size table Models of E3–E2 ∼ Ub complexes suggest a basis for activation Although our affinity measurements do not support enhanced interaction between any of the PCGF E3s and charged E2, we nevertheless found ubiquitin recognition by E3 a compelling mechanism to explore. Structures of RING E3s in complex with charged UbcH5-family E2s reveal a consistent arrangement of the E2, the RING and Ub [30] , [31] , [33] , [34] , [35] ( Fig. 3 ; Supplementary Fig. 5 ). For dimeric RING E3s, one (proximal) RING binds the E2, while an aromatic residue (in some cases bolstered by an arginine) from the E2 distal RING interacts with Ub [30] , [33] ( Fig. 3a,b ). In the case of the monomeric p-CBL-B ligase, a phosphorylated tyrosine mediates interactions with Ub [34] ( Fig. 3c ). Essentially, RING E3s shift the ensemble population of E2 ∼ Ub to a more restricted (closed) state, increasing reactivity towards substrate lysine [30] , [31] , [32] . The conservation of this mechanism is notable, and it seemed likely to be applicable to other RING–UbcH5 pairs. Accordingly, we generated models of PCGF and other E3s bound to Ub-charged UbcH5. A model for cIAP2 ( Fig. 3d ) predicts Phe602 to contact Ub, consistent with studies demonstrating the importance of this residue for E3 activity [45] . Likewise, the MDM2–MDMX model ( Fig. 3e ) places MDMX Phe488 in the Ub interface, again consistent with mutagenesis results [46] . The concordance between models and other studies suggests that the mode of Ub recognition is indeed general. The corresponding models for PCGF5 and PCGF4 complexes ( Fig. 3f,g ) suggest features reminiscent of both the homodimeric RING and p-CBL-B structures. Like RNF4 and BIRC7, the Ub contact surface includes residues from the E2-distal RING, in this case from the PCGF subunit helix α3, and like CBL-B, the primary contact is charged rather than aromatic (see also the recent RNF38 example [35] ). For both PCGFs, there is a negatively charged residue roughly in the position of the phosphotyrosine of p-CBL-B (see E77 in Fig. 3f and D77 in Fig. 3g ). In addition, a second polar residue on the same surface of α3 is in proximity to Ub (N73 and K73 for PCGF5 and PCGF4, respectively). Figure 3: Interactions between ubiquitin (Ub) and E3. ( a – c ) Close-up views of the E3-Ub interface from previously reported crystal structures. For the homodimeric E3s, Ub (orange) makes contacts with the E2-distal monomer (green). E3 residues shown in cyan mediate interactions with Ub. For the monomeric CBL-B, phosphorylation mediates the E3-Ub interaction. ( d – g ) Previous crystal structures were combined using structural overlays to generate models of E3–E2 ∼ Ub complexes. A close-up view of the modelled E3-Ub interface is shown in each case (with RING monomers coloured as at top). Residues from the E3 that are expected to contact Ub are shown in cyan. ( d ) Model of cIAP2–UbcH5 ∼ Ub complex. The experimental structure of cIAP2–UbcH5b (3EB6 (ref. 45 )) was overlaid with that of BIRC7–UbcH5b ∼ Ub (4AUQ [30] ) by aligning the E2s. ( e ) Model of MDM2–MDMX–UbcH5 ∼ Ub generated by aligning the MDM2 monomer from the MDM2–MDMX structure (2VJE [70] ) with the E2 proximal BIRC7 monomer from 4AUQ [30] . ( f , g ) Models of PCGF5– and PCGF4–RING1B-UbcH5 ∼ Ub generated by overlaying the structure reported here ( f ) or 3RPG ( g ) with 4AUQ [30] by aligning the E2s. Full size image Multiple sequence alignment ( Supplementary Fig. 6 ) reveals that residues in helix α3 are nearly invariant across species for a given PCGF family member. Intriguingly, the identities of two putative Ub contact residues described above allow a separation of the low- and high-activity groups ( Fig. 4a ; Supplementary Fig. 6 ). In particular, all low-activity PCGFs except for Psc share the equivalent of K73 and D77 from human PCGF4. The analogous residues in the high-activity group are generally arginine and aspartic acid (the N/E combination seen in PCGF5 orthologues is the exception; Fig. 4a ). To test whether these sequence differences were functionally important, we introduced into PCGF4 PCGF high activity residues and screened initially in the auto-ubiquitination assay. Both PCGF4 mutants (K73N/D77E; P4 M and K73R; P4 KR) support higher activity than WT PCGF4 ( Fig. 4b ). Interestingly, the function of these amino acids appears to be modular, as introduction of the three residue combinations of human into the more divergent Drosophila Psc yields the appropriate high- or low-activity E3 ( Fig. 4c ). 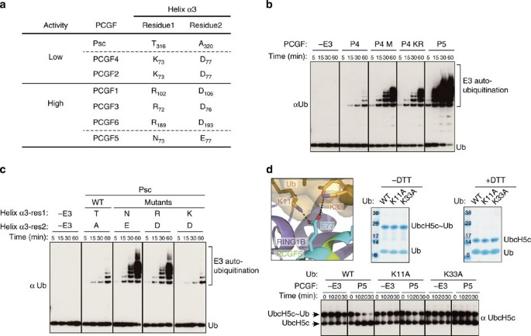Figure 4: PCGF helix α3 residues strongly modulate E3 ligase activity as monitored by western blot. (a) Identities of putative Ub contact residues from helix α3 of the different PCGFs. (b) Auto-ubiquitination catalysed by PCGF4–RING1B mutant complexes in which the two helix α3 residues are taken from the high-activity group PCGFs. ‘P4 M’ denotes the PCGF4 mutant with PCGF5 α3 residues, while ‘P4 KR’ incorporates the K73R mutation (as present in PCGFs 1, 3 and 6). (c) Introduction of human helix α3 residue pairs into Psc of the Psc–Sce complex. Auto-ubiquitination activity tracks with the high or low activity of the corresponding human complex (Fig. 1b). (d) A structural model suggests E3 recognition of ubiquitin lysine residues. Top left: potential interaction between PCGF5 E77 (cyan) and Ub K11 and K33. Bottom: discharge of E2∼Ub (wt or mutants) to lysine catalysed by RING1B–PCGF5. Substrate and product were detected with α-UbcH5c antibody instead of α-Ub to avoid potential differences in detection of different Ub mutants by the latter. Note that the α-UbcH5c antibody used here detects uncharged E2 much more strongly than charged E2. The prominent E2 band at the earliest time point represents only a trace amount of uncharged E2 in the substrate as indicated by Coomassie staining (shown at top center and right). Figure 4: PCGF helix α3 residues strongly modulate E3 ligase activity as monitored by western blot. ( a ) Identities of putative Ub contact residues from helix α3 of the different PCGFs. ( b ) Auto-ubiquitination catalysed by PCGF4–RING1B mutant complexes in which the two helix α3 residues are taken from the high-activity group PCGFs. ‘P4 M’ denotes the PCGF4 mutant with PCGF5 α3 residues, while ‘P4 KR’ incorporates the K73R mutation (as present in PCGFs 1, 3 and 6). ( c ) Introduction of human helix α3 residue pairs into Psc of the Psc–Sce complex. Auto-ubiquitination activity tracks with the high or low activity of the corresponding human complex ( Fig. 1b ). ( d ) A structural model suggests E3 recognition of ubiquitin lysine residues. Top left: potential interaction between PCGF5 E77 (cyan) and Ub K11 and K33. Bottom: discharge of E2 ∼ Ub (wt or mutants) to lysine catalysed by RING1B–PCGF5. Substrate and product were detected with α-UbcH5c antibody instead of α-Ub to avoid potential differences in detection of different Ub mutants by the latter. Note that the α-UbcH5c antibody used here detects uncharged E2 much more strongly than charged E2. The prominent E2 band at the earliest time point represents only a trace amount of uncharged E2 in the substrate as indicated by Coomassie staining (shown at top center and right). Full size image In our structural model and in a similar published model [30] , PCGF4 K73 clashes sterically with Ub, which implies either that K73 must move to allow Ub to bind in an activated conformation or that Ub adopts a less optimal position during transfer ( Fig. 3 ; Supplementary Fig. 7a ). Either of these could provide an energy barrier, slowing transfer catalysed by PCGF4. Conversely, the PCGF5 interface appears complementary, and the model suggests that PCGF5 E77 would interact with Ub K11 and K33 ( Fig. 3 ; Supplementary Fig. 7b ). Therefore, we tested whether PCGF5–RING1B could catalyse discharge of Ub(K11A) and Ub(K33A) from UbcH5c to solution lysine. (The E2 discharge assay, unlike the auto-ubiquitination assay, does not rely on the formation of poly-Ub chains and is therefore more appropriate for evaluation of Ub lysine mutants. We used α-UbcH5c antibody instead of α-ubiquitin to ensure uniform detection of substrate and product.) As predicted from the model, the E2 discharge rate was greatly diminished for both Ub lysine mutants compared with wild-type (WT) UbcH5c ∼ Ub ( Fig. 4d ). We found a very similar effect on discharge rates of these E2 ∼ Ub mutants by PCGF6–RING1B, in which the critical α3 residue is aspartic acid instead of glutamic acid ( Supplementary Fig. 7c ). Thus, despite the lack of Ub enhancement of E2 affinity for the PCGF E3s, the collective results demonstrate the importance of a PCGF-Ub interface in a similar position to that characterized structurally for other RING E3s. In the case of the PCGF ligases, it would seem that this interaction occurs as a high-energy intermediate that is not significantly populated in the ground state but is nevertheless important in catalysis. Canonical PRC1 E3s are optimized for poor intrinsic activity The experiments above revealed the importance of two PCGF α3 Ub contact residues in determining the level of E3 activity. However, the activities of PCGF4 mutants were still short of the full activation seen for RING1B–PCGF5 and the other high-activity PCGF E3s. We therefore compared mutation of PCGF4 α3 residues (P4 M; Fig. 4b ), the partially activating N-terminal chimera described above (P4 S; Fig. 2c ), and the combination of the two (P4 SM; Fig. 5a ). Introducing the two changes together increases the ligase activity of the mutant PCGF4 complex to a level close to that of the RING1B–PCGF5 complex in both auto-ubiquitination ( Fig. 5a ) and E2 discharge assays ( Fig. 5b ). Comparison of k 2 values determined from the FP-monitored E2 discharge assay reveals P4 SM to be 14-fold more active than PCGF4 (and more active than any of the PCGF high activity variants; Fig. 5c ; Table 1 ). The reciprocal changes in PCGF5 greatly reduced ligase activity compared with the WT complex (11-fold decrease in k 2 for P5 SM; Supplementary Fig. 8 ; Table 1 ). We conclude that a non-optimal Ub contact surface and an allosteric effect from the N-terminal dimerization interface together tightly regulate the low-activity PCGFs. 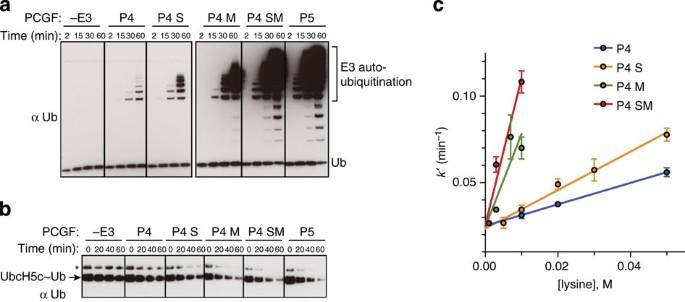Figure 5: Re-engineering the PCGF4–RING1B ligase for high activity. (a,b) N-terminal swap with PCGF5 (P4 S;Fig. 2c) and helix α3 mutations (P4 M;Fig. 4) were evaluated individually or combined (P4 SM) in the wild-type background of PCGF4. E3 activity of the RING1B complex was assessed in the auto-ubiquitination assay (a) or the E2 discharge assay (b) as visualized by western blot. ‘*’ marks a band that appears to be UbcH5c conjugated to diUb. (c). E2 discharge quantified by FP. Data are plotted as pseudo first-order rate constants (k′±s.d.) versus lysine concentration. Averages were determined from duplicate measurements for all PCGF4 variants. Second-order rate constants (slopes of the linear fits shown) are reported inTable 1. Figure 5: Re-engineering the PCGF4–RING1B ligase for high activity. ( a , b ) N-terminal swap with PCGF5 (P4 S; Fig. 2c ) and helix α3 mutations (P4 M; Fig. 4 ) were evaluated individually or combined (P4 SM) in the wild-type background of PCGF4. E3 activity of the RING1B complex was assessed in the auto-ubiquitination assay ( a ) or the E2 discharge assay ( b ) as visualized by western blot. ‘*’ marks a band that appears to be UbcH5c conjugated to diUb. ( c ). E2 discharge quantified by FP. Data are plotted as pseudo first-order rate constants (k′±s.d.) versus lysine concentration. Averages were determined from duplicate measurements for all PCGF4 variants. Second-order rate constants (slopes of the linear fits shown) are reported in Table 1 . Full size image The six PCGF E3s all recognize the H2A/H2B acidic patch The E3 ligase activity of BMI1 (PCGF4)–RING1B has been characterized extensively in published biochemical studies [8] , [9] , [37] , [38] , [47] . Both intact PRC1 purified from cells and the minimal RING–RING constructs of PCGF4–RING1B we employ here monoubiquitinate Histone H2A at K118/K119, a reaction requiring intact nucleosome as a substrate [37] , [38] . That the RING domains alone constitute a biochemically active E3 with the same site specificity as the intact complex strongly implied that the RINGs themselves were capable of nucleosome recognition [37] , [38] (now a broader phenomenon recently reviewed in ref. 48 ). We found previously that basic surface patches on PCGF4- and RING1B-mediated binding to short DNA duplexes and that mutation of these basic residues reduced or eliminated ubiquitination activity [37] . This suggested that nucleosomal DNA provided a scaffold for E3 recruitment and orientation [37] . However, the basic residues of PCGF4 we associated with DNA binding and full H2A ubiquitination activity, K62 and R64 (ref. 37 ), are conserved only in PCGF2 (MEL-18) but not in the other four human PCGFs (1, 3, 5 and 6; Supplementary Fig. 1a ). To establish whether each of the six core RING–RING complexes was an active H2A ligase, we evaluated ubiquitination activity using a reconstituted mononucleosome substrate. We found that although four PCGF complexes lacked an important substrate interaction feature of PCGF4, these ‘non-canonical’ RING–RING heterodimers nevertheless catalysed H2A ubiquitination ( Fig. 6a ). Furthermore, as previously found for PCGF4–RING1B [37] , [38] , each required an intact nucleosome substrate ( Fig. 6a ). It is notable that the activities of the six complexes appear much more similar in this assay than they do when evaluated for intrinsic E3 activity. This observation, coupled with the absence in the non-canonical ligases of the basic patch present on PCGF4, suggested that the canonical and non-canonical PCGF complexes might recognize nucleosome differently. 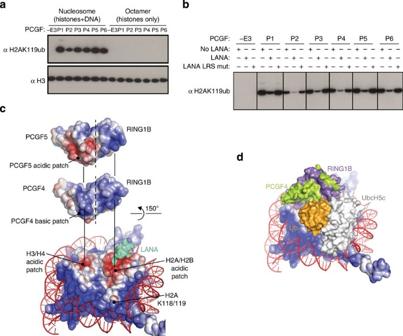Figure 6: Recognition of the nucleosome by the RING1B–PCGF–UbcH5c∼Ub complexes. (a) Ubiquitination of Histone H2A in mononucleosomes (left) or ‘octamers’ (right; see Methods) by the different RING1B–PCGF E3s, Top: western blot using α-H2A K119ub antibody, Bottom: western blot using α-H3 antibody (b) LANA peptide inhibition of RING1B–PCGF ubiquitination of Histone H2A. Each RING1B–PCGF was tested in the absence of LANA peptide, or in the presence of wild-type or non-binding (LRS) mutant peptide; see Methods for sequences). Product was detected by western blot using α-H2A K119ub antibody. (c) Structure of the nucleosome core particle at left showing location of acidic surface patches (H2A E92 and surrounding residues form the major patch; the smaller patch is formed by H3 E73, H3 D77 and H4 D24), location of the site of ubiquitination of H2A by PCGF ligases, and bound LANA peptide in cyan (PDB: 1ZLA51). The location of charged surface patches on RING1B–PCGF RING dimers is shown above. (d) Model of the RING1B–PCGF4–UbcH5c nucleosome complex with Ub in a transfer competent position. The model is based on the required proximity of the E2 active site cysteine and H2A K118/119, as well as the requirement of the H2A acidic patch for RING1B–PCGF ligase activity49and the LANA peptide inhibition data shown inb. RING1B is positioned over the H2A acidic patch. (Note that this is not a docked model, thus detailed interactions are not predicted, only the approximate positions of the various proteins. An experimental structure has been reported recently52for this E2-E3-substrate complex without ubiquitin present.) Electrostatic potential molecular surface of the histone octamer shown incanddwas generated from the structure of the nucleosome core particle (PDB: 1AOI71) using the Adaptive Poisson-Boltzman Solver (APBS) plugin in PyMOL (Schrödinger LLC), contoured to ±4.0 kT/e. Figure 6: Recognition of the nucleosome by the RING1B–PCGF–UbcH5c ∼ Ub complexes. ( a ) Ubiquitination of Histone H2A in mononucleosomes (left) or ‘octamers’ (right; see Methods) by the different RING1B–PCGF E3s, Top: western blot using α-H2A K119ub antibody, Bottom: western blot using α-H3 antibody ( b ) LANA peptide inhibition of RING1B–PCGF ubiquitination of Histone H2A. Each RING1B–PCGF was tested in the absence of LANA peptide, or in the presence of wild-type or non-binding (LRS) mutant peptide; see Methods for sequences). Product was detected by western blot using α-H2A K119ub antibody. ( c ) Structure of the nucleosome core particle at left showing location of acidic surface patches (H2A E92 and surrounding residues form the major patch; the smaller patch is formed by H3 E73, H3 D77 and H4 D24), location of the site of ubiquitination of H2A by PCGF ligases, and bound LANA peptide in cyan (PDB: 1ZLA [51] ). The location of charged surface patches on RING1B–PCGF RING dimers is shown above. ( d ) Model of the RING1B–PCGF4–UbcH5c nucleosome complex with Ub in a transfer competent position. The model is based on the required proximity of the E2 active site cysteine and H2A K118/119, as well as the requirement of the H2A acidic patch for RING1B–PCGF ligase activity [49] and the LANA peptide inhibition data shown in b . RING1B is positioned over the H2A acidic patch. (Note that this is not a docked model, thus detailed interactions are not predicted, only the approximate positions of the various proteins. An experimental structure has been reported recently [52] for this E2-E3-substrate complex without ubiquitin present.) Electrostatic potential molecular surface of the histone octamer shown in c and d was generated from the structure of the nucleosome core particle (PDB: 1AOI [71] ) using the Adaptive Poisson-Boltzman Solver (APBS) plugin in PyMOL (Schrödinger LLC), contoured to ±4.0 kT/e. Full size image Significant insight into nucleosome recognition is gained from the recent finding that ubiquitination by PCGF4–RING1B requires an acidic patch present on Histone H2A (E92) [49] that is also a required recognition element for the ligase RNF168 (refs 49 , 50 ). The H2A acidic patch is also the binding site for a 22 amino-acid peptide from the Kaposi’s sarcoma-associated herpes virus protein LANA [51] , and binding of the LANA peptide to nucleosome blocks RNF168 ubiquitination of H2A K13/K15 (refs 49 , 50 ). To verify and extend the conclusion that PCGF4–RING1B recognizes the H2A acidic patch, we tested whether the LANA peptide inhibits ubiquitination of nucleosome by the six PCGF–RING1B complexes ( Fig. 6b ). Activity of all the six complexes is blocked by added LANA peptide but not by control peptide (LANA LRS mutant [51] ), consistent with the idea that all the PCGF ligases recognize the nucleosome through the H2A acidic patch. Thus, our earlier association of DNA binding with the mode of nucleosome recognition [37] is incorrect. It remains possible that DNA binding could contribute to other aspects of canonical PRC1 function, for example, to chromatin compaction. The finding of LANA peptide inhibition may be incorporated into a model for E2–E3 nucleosome interaction. Positioning the basic residues of the shared E3 subunit RING1B that are critical for activity (K97 and R98 (ref. 37 )) to interact with H2A E92 and overlap the LANA peptide-binding site (H2A/H2B acidic patch; Fig. 6c ) places the relevant basic patch of PCGF4 (K62 and R64 (ref. 37 )) near the H3/H4 acidic patch ( Fig. 6c ). (This arrangement is consistent with a crystal structure of the PCGF4–RING1B–UbcH5c complex bound to nucleosome published during review of our manuscript [52] . In particular, direct interactions were found between H2A E92 and RING1B R98 and between H3 D77 and PCGF4 R64.) In contrast, the analogous surface of PCGF5 is acidic and therefore appears less complementary ( Fig. 6c ). Interaction with both nucleosome acidic patches is consistent with the PCGF–RING1B requirement for an intact nucleosome substrate. In contrast, the monomeric E3 RNF168 (that interacts predominantly with H2A) can selectively ubiquitinate H2A–H2B dimer [50] . Dual substrate recognition important for H2A ubiquitination The consistent inhibition with LANA peptide suggests that all the six PCGF–RING1B complexes occupy a similar footprint on the nucleosome substrate. Given that, we wondered whether the much greater intrinsic E3 activity of the PCGF5–RING1B might result in faster H2A ubiquitination, evident perhaps at an earlier stage of the reaction. To evaluate this, we monitored H2A K119ub formation by PCGF4–RING1B and PCGF5–RING1B complexes over time ( Fig. 7a ). Surprisingly, no large difference in reaction rate was apparent. To investigate product formation quantitatively, we used Alexa Fluor 488-labelled Ub as a substrate, then imaged and quantified the product bands from gels. This allowed us to test the effects of mutations affecting intrinsic E3 activity (combination mutants ‘SM’, previously shown in Fig. 5 and Supplementary Fig. 8 ) and mutations in the PCGF basic patch (designated ‘BP’, Fig. 7b ) in the context of the nucleosome reaction. For PCGF4–RING1B, the E3-activating mutations greatly increase the rate of nucleosome ubiquitination (P4 SM; Fig. 7c ; Supplementary Fig. 9a,b ). In contrast, the mutation of two PCGF4 basic patch residues to PCGF5 counterparts (K62E/R64N; Fig. 7b ) markedly decreases the rate of H2A K119ub formation (P4 BP; Fig. 7d ) without any apparent effect on E2 discharge rate ( Supplementary Fig. 9c,d ; Table 1 ). The combination of BP and SM mutations (P4 SM+BP) results in a rate similar to WT ( Fig. 7c ), suggesting that these surfaces contribute independently to the overall reaction. A similar pattern was observed for PCGF5 mutants ( Fig. 7d ; Supplementary Fig. 9a,b ), although in the nucleosome assay, the P5 SM mutant is not fully inactivating. Notably, the rate of the PCGF5-catalysed reaction can be greatly increased by providing PCGF5 with a PCGF4-like basic patch. Taken together, these data support cooperation between E3 recognition of both ubiquitin and nucleosome in promoting H2A ubiquitination. It remains to be determined in detail how other PRC1 complex components, or regulatory mechanisms such as activating phosphorylation of PCGF proteins [53] , [54] or inactivating phosphorylation of RING1B within PRC1.5 (ref. 55 ), influence E3 ligase activity of canonical and non-canonical PRC1. 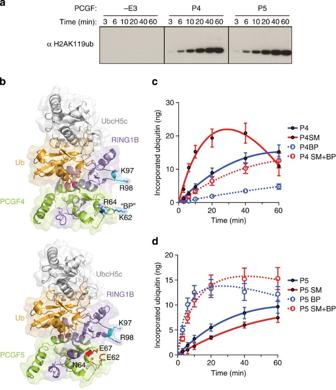Figure 7: Intrinsic E3 activity and nucleosome recognition each contribute to the rate of Histone H2A ubiquitination. (a) Nucleosome ubiquitination catalysed by PCGF4 and PCGF5 at the indicated time points. (b) Identities and positions of residues important for nucleosome ubiquitination. RING1B K97 and R98, as well as PCGF4 K62 and R64 (shown at top) were shown previously to be functionally important37. The residues in PCGF5 at positions equivalent to K62 and R64 are E62 and N64. There is an additional charged residue E67 that contributes to the acidic surface patch of PCGF5. (c,d) Mutants of PCGF4 and PCGF5 evaluated in a quantitative nucleosome ubiquitination assay. Incorporation of Alexa Fluor 488-tagged ubiquitin into H2A K119ub1 was quantified as described in Methods. Reactions were run in three independent experiments and data presented as mean value±s.e.m. (c) Wild-type complex (P4) is compared with the most active chimeric mutant shown inFig. 5(P4 SM), a mutant exchanging basic patch residues for those residues present in PCGF5 (P4 BP≡PCGF4 K62E/R64N), and a combination of P4 SM and P4 BP (P4 SM+BP). For the fastest reaction (P4 SM), product disappears at later time points because of conversion to a second product that appears to be H2Aub2 (seeSupplementary Fig. 9a). (d) H2A K119ub1 formation catalysed by PCGF5 mutant complexes analogous to the PCGF4 variants shown inc. In the case of the P5 BP mutant, the flanking acidic residue E67 was also changed to the corresponding PCGF4 amino acid (E62K/N64R/E67L) to fully switch the charged patch from acidic to basic. Figure 7: Intrinsic E3 activity and nucleosome recognition each contribute to the rate of Histone H2A ubiquitination. ( a ) Nucleosome ubiquitination catalysed by PCGF4 and PCGF5 at the indicated time points. ( b ) Identities and positions of residues important for nucleosome ubiquitination. RING1B K97 and R98, as well as PCGF4 K62 and R64 (shown at top) were shown previously to be functionally important [37] . The residues in PCGF5 at positions equivalent to K62 and R64 are E62 and N64. There is an additional charged residue E67 that contributes to the acidic surface patch of PCGF5. ( c , d ) Mutants of PCGF4 and PCGF5 evaluated in a quantitative nucleosome ubiquitination assay. Incorporation of Alexa Fluor 488-tagged ubiquitin into H2A K119ub1 was quantified as described in Methods. Reactions were run in three independent experiments and data presented as mean value±s.e.m. ( c ) Wild-type complex (P4) is compared with the most active chimeric mutant shown in Fig. 5 (P4 SM), a mutant exchanging basic patch residues for those residues present in PCGF5 (P4 BP≡PCGF4 K62E/R64N), and a combination of P4 SM and P4 BP (P4 SM+BP). For the fastest reaction (P4 SM), product disappears at later time points because of conversion to a second product that appears to be H2Aub2 (see Supplementary Fig. 9a ). ( d ) H2A K119ub1 formation catalysed by PCGF5 mutant complexes analogous to the PCGF4 variants shown in c . In the case of the P5 BP mutant, the flanking acidic residue E67 was also changed to the corresponding PCGF4 amino acid (E62K/N64R/E67L) to fully switch the charged patch from acidic to basic. Full size image The PCGF–RING1 ligases provide an advantageous experimental system in which to evaluate the regulatory potential of different RING domains on a common RING E3 binding partner. We find that a non-E2 contacting RING can not only activate its partner but also keep it tightly in check. This inhibition is mechanistically distinct from autoinhibition in the RING-in-between-RING class of E3 ligases, such as Parkin (recently reviewed in ref. 56 ). In RING-in-between-RING ligases, a flanking domain blocks access to the catalytic cysteine, while in the PCGF RING heterodimers, the level of activity is intrinsic to the catalytic core. Given the large number of potential RING–RING interactions emerging from screens and the frequent involvement of non-E2-binding RING proteins [57] , many combinations may serve to fine tune E3 output. In the human PCGF family, we find that the two members, PCGF4/BMI1 and PCGF2/Mel-18, support only low-level intrinsic RING1B activity in auto-ubiquitination or E2 discharge assays. This effect can be attributed largely to a pair of PCGF2/4 helix α3 residues (K73 and D77) predicted to interact with ubiquitin during catalysis. The most common difference in the more active PCGFs is K73R, and this substitution is highly activating when introduced into PCGF4 ( Fig. 4b ). Intriguingly, a recent (and comprehensive) survey of salt bridging in protein crystal structures suggests an explanation: the K i , D i +4 intrahelical residue pair was found to have by far the greatest propensity to form a salt bridge of any combination evaluated [58] (approximately sevenfold more likely than R i , D i +4 , predicting ∼ 1.2 kcal mol −1 greater stability for the K i , D i +4 interaction). In agreement with the general trend, we observe clearly the K73–D77 salt bridge in all published structures of RING1B–PCGF4 ( Supplementary Fig. 10 ). We suggest that the salt bridge both interferes sterically with the close approach of ubiquitin and limits the capacity of D77 to engage in alternative interactions with Ub K11 and K33. The ligase may remain inactive until a favourable, complementary interaction between E3–E2 ∼ Ub and nucleosome substrate overcomes the energy barrier imposed by the PCGF surface salt bridge. Such a mechanism could enhance ligase fidelity by preventing premature Ub discharge to an inappropriate substrate. A related advantage to specific substrate activation of Ub transfer is that it may disfavour chain extension after initial monoubiquitination. The potential importance of faithful H2A monoubiquitination is underscored by the recent discovery of ‘readers’ of this modification [29] , [59] , [60] , [61] . Very recently, compelling evidence has emerged supporting differential cellular H2A ubiquitination activity for canonical and non-canonical PRC1 (ref. 29 ). Intact canonical PRC1 (PCGF2 or PCGF4) was directed to a defined chromatin domain through fusion to a sequence-specific DNA-binding protein TetR (or by selective deposition of H3K27me3) but failed to ubiquitinate H2A K119 despite recruitment of RING1B to the domain. In contrast, TetR fusions of non-canonical PCGFs 1, 3 and 5 readily produced H2A K119ub. Interestingly, activity of PCGF4–RING1B could be seen when only the core RING–RING heterodimer was fused to TetR, suggesting that the intact complex is inhibited by a component other than the RING domains [29] ; it is possible, however, that canonical PRC1 is more dependent than non-canonical PRC1 on binding in a highly specific orientation to facilitate catalysis. Enforced proximity may be sufficient to allow the intrinsically more active non-canonical ligases to achieve an acceptable interaction with substrate. Overall, the results support a high degree of regulation of PRC1 ubiquitination activity consistent with the differences we see between canonical and non-canonical PCGF–RING1B complexes. For non-canonical PRC1, it may be unimportant, perhaps even deleterious, to restrict activity in the manner seen for canonical PRC1 E3s. For example, non-canonical PRC1 ligases could have an expanded list of client substrates and if so, it might explain why they have not maintained optimal binding to the nucleosome surface. The requirement for non-canonical PRC1 complexes in ES cell proliferation [62] , retroviral repression [63] , and regulation of metabolic genes and cell cycle progression [25] may be consistent with a need for greater flexibility (faster intrinsic rate, lower affinity for substrate) compared with the action of canonical PRC1 during development (where precision may be of paramount importance). The recent rapid progress in this area suggests that important elements of PCGF–RING1 E3 ligase function and regulation may yet be discovered. Expression and purification of RING1–PCGF complexes The RING domain of each PCGF protein was cloned into the pET24-b vector (EMD Millipore) as previously described [37] , resulting in a construct expressing the PCGF with a C-terminal His 6 tag (non-cleavable). The human PCGF RING domains spanned the following residues ( Fig. 1a ): PCGF1 (1–138); PCGF2 (1–109); PCGF3 (1–108); PCGF4 (1–109); PCGF5 (1–109); and PCGF6 (101–225). An analogous plasmid was constructed to express the RING domain from the D. melanogaster PCGF orthologue Psc (UniProt: P35820, residues 242–353). Human RING1B (1–116), RING1A (1–113) and D. melanogaster Sce/dRING (1–111) were cloned into pGEX6P-1 (GE Healthcare). The resulting constructs express the RING1 variants with an N-terminal GST tag and a PreScission protease cleavage site. RING1–PCGF complexes were expressed in Escherichia coli Rosetta 2 (Novagen). Cells were grown to D 600 nm of ∼ 0.9 in LB media at 37 °C, treated with 0.5 mM isopropyl-β- D -thiogalactoside (IPTG) to induce expression and shaken overnight at 16 °C. Cell pellets were resuspended and lysed in buffer containing 50 mM Tris pH 7.5, 150 mM NaCl, 20 mM imidazole, 1 mM dithiothreitol (DTT) and supplemented with EDTA-free Complete protease inhibitor tablets (Roche). The RING1–PCGF complexes were purified first using Ni NTA Superflow resin (Qiagen). After flowing lysate over the Ni NTA resin, the resin was washed with 50 mM Tris pH 7.5, 150 mM NaCl, 20 mM imidazole and 1 mM DTT. The fraction eluted from the Ni NTA resin using 50 mM Tris pH 7.5, 150 mM NaCl, 250 mM imidazole and 1 mM DTT was applied directly onto Glutathione Sepharose 4B resin (GS4B, GE Healthcare). For GST-tagged versions of the complex used in auto-ubiquitination assays and binding studies, the proteins were eluted from the GS4B resin with 50 mM Tris pH 7.5, 150 mM NaCl, 1 mM DTT and 10 mM glutathione and subjected to size-exclusion chromatography (SEC) on a Superdex 200 column equilibrated with 20 mM Tris pH 7.5, 150 mM NaCl and 1 mM DTT. For the nucleosome ubiquitination and E2 discharge assays, the RING1–PCGF complexes were not eluted from the GS4B resin, but were instead subjected to on-column tag cleavage using PreScission protease (GE Healthcare) according to the manufacturer’s protocol, at 4 °C overnight. Following cleavage of the GST tag, proteins were subjected to SEC on Superdex 200 as described above. All proteins and complexes were pooled from a single SEC peak of expected molecular weight, and purity (>95%) was confimed by SDS–polyacrylamide gel electrophoresis. Gels showing purities of key complexes are shown in Supplementary Fig. 11 . Proteins were concentrated as necessary using Amicon Ultra centrifugal filter units (Millipore), stored in the SEC buffer (unless specified), and concentration was determined using A 280 (NanoDrop, Thermo Scientific) with extinction coefficients calculated using the ProtParam tool (ExPASy, http://web.expasy.org/protparam/ ). Expression and purification of UbcH5c and ubiquitin UbcH5c was cloned into pGEX6P-1 (GE Healthcare) as described previously [37] and expressed in E. coli Rosetta 2 or Rosetta 2 pLysS cells (Novagen). Cells were grown to D 600 nm of ∼ 0.9 in LB media at 37 °C, treated with 0.5 mM IPTG to induce expression, and shaken overnight at 16 °C. Cell pellets were resuspended and lysed in buffer containing 50 mM Tris pH 7.5, 200 mM NaCl, 20 mM imidazole and 1 mM DTT and supplemented with EDTA-free Complete protease inhibitor tablets (Roche). UbcH5c was first purified over GS4B (GE Healthcare) followed by on-column tag cleavage with PreScission protease (GE Healthcare) using the GE Healthcare protocol, at 4 °C overnight. This was followed by cation-exchange chromatography using a NaCl gradient on a HiTrap SP HP column (GE Healthcare). The buffer was then exchanged using Zeba desalting columns (Thermo Scientific) to 50 mM HEPES pH 7.2, 100 mM NaCl and 1 mM DTT for storage. For purification of UbcH5c(S22R/C85K), the protein was run over a Superdex 200 equilibrated with 20 mM Tris pH 7.5, 150 mM NaCl and 1 mM DTT. Ubiquitin was cloned into pET15b (EMD Millipore) to yield a coding sequence with a N-terminal His 6 tag followed by a thrombin cleavage site and ubiquitin. Ubiquitin was expressed in BL21 (DE3). Cells were grown in TB+1% glycerol, 100 mM MOPS pH 7.3 to an D 600 of >1.5. Flasks were then cooled at 16 °C for ∼ 45 min, and cells were treated with 0.5 mM IPTG to induce expression, then shaken overnight at 16 °C. Cell pellets were resuspended and lysed in buffer containing 40 mM Tris pH 8.0 and 300 mM NaCl and supplemented with EDTA-free Complete protease inhibitor tablets (Roche). Ubiquitin was purified over Ni NTA Superflow resin (Qiagen). After loading the lysate, the resin was washed with 20 mM Tris pH 8.0, 1 M NaCl and 20 mM imidazole. The protein was eluted from resin with 20 mM Tris pH 8.0, 500 mM NaCl and 250 mM imidazole. The eluted product was applied to a Superdex 200 column equilibrated with 20 mM Tris pH 7.5, 150 mM NaCl and 1 mM DTT. Alexa Fluor 488-conjugated ubiquitin was prepared from ubiquitin tagged at the N terminus with the sequence CGS. CGS ubiquitin (170 μM in 50 mM HEPES, pH 7.2, 150 mM NaCl) was treated with a fourfold molar excess of Alexa Fluor 488 C5 maleimide (A10254; Life Technologies) by the addition of an appropriate volume from a 10 mM DMSO stock. After 3-h reaction at room temperature, reaction was quenched by the addition of 10 mM DTT, and the ubiquitin was desalted on a PD-10 column (GE Healthcare) to remove the excess dye. Alexa-488 ubiquitin was concentrated using an Amicon Ultra centrifugal filter unit (Millipore) and stored until use at −80 °C. BODIPY-FL-conjugated ubiquitin was prepared from CGS ubiquitin in an analogous manner. CGS ubiquitin (112 μM) was treated with 450 μM BODIPY-FL maleimide (B-10250; Life Technologies) and isolated as described above. The conjugate was subjected to analysis by LC-MS (Agilent Infinity 1260 high-performance liquid chromatography coupled with an Agilent 6224 mass analyser). Proteins were separated on a PRLP-S reverse-phase column with a gradient of acetonitrile in water (0.05% trifluoroacetic acid), and data were analysed using the Mass Hunter software (Agilent). Labelling of CGS -ubiquitin with BODIPY-FL was determined to be complete and stoichiometric (1:1). General procedures for electrophoresis and western blotting The quenched reaction products from assays were resolved on 4–12% NuPAGE Bis-Tris gels run in MES buffer (Life Technologies) and were transferred onto nitrocellulose membranes using the iBlot device (Life Technologies). The membrane was blocked with 5% nonfat milk (Bio-Rad) prepared in 1 × PBS, 0.05% Tween-20 (with rocking at room temperature, 1 h) All antibody dilutions were made using this solution. Membranes were probed with α-ubiquitin-horseradish peroxidise (HRP; P4D1, Santa Cruz Biotechnology) at 1:2,000 dilution (rocking at room temperature, 1 h). This was followed by two 10-min washes with 1 × PBS, 0.05% Tween-20 (rocking at room temperature). Bands were visualized using ECL Prime (GE Healthcare). For the E2 discharge assay with ubiquitin mutants, the membrane was probed with α-UbcH5c (Cell Signaling, #4330) at 1:5,000 dilution (rocking at room temperature, 1 h). This was followed by two 10-min washes with 1 × PBS, 0.05% Tween-20 and incubation with α-rabbit-HRP (Cell Signaling, #7074) at 1:3,000 dilution (rocking at room temperature, 45 min). The membrane was washed as above, and bands were visualized using ECL Prime (GE Healthcare). Auto-ubiquitination assays His 6 -E1 (0.5 μM; Boston Biochem), 2.5 μM UbcH5c, 2 μM GST–RING1–PCGF and 10 μM His 6 -Ub (Boston Biochem) were incubated in 50 mM HEPES pH 8.0, 10 mM ATP and 10 mM MgCl 2 at room temperature for the time specified. Reactions were quenched in LDS sample buffer containing DTT. Electrophoresis and western blotting were performed as described above. E2 discharge assay UbcH5c was charged with ubiquitin (to form a pool of UbcH5c ∼ Ub) using 0.75 μM His 6 -E1 (Boston Biochem), 40 μM UbcH5c and 80 μM His 6 -Ub (Boston Biochem) in a buffer containing 50 mM HEPES pH 8.0, 10 mM MgCl 2 , 50 mM NaCl and 0.2 mM DTT, for 30 min at 35 °C. Charging was stopped by adding 50 mM EDTA and desalting the proteins into a final buffer containing 50 mM HEPES pH 7.2 and 50 mM NaCl using 0.5 ml Zeba spin desalting columns (Thermo Scientific). Discharge of the UbcH5c ∼ Ub pool was carried out by the addition of each RING1–PCGF (5 μM final) to ∼ 10 μM desalted UbcH5c ∼ Ub in the presence of 10 mM lysine at room temperature. At various time points, the discharge reaction was quenched with LDS sample buffer. Electrophoresis and western blotting were performed as described above. E2 discharge monitored by fluorescence polarization UbcH5c was charged with BODIPY-FL-labelled ubiquitin in a solution containing 5 μM E1 (Boston Biochem), 417 μM UbcH5c, 513 μM BODIPY-FL ubiquitin (see above), 10 mM ATP, 10 mM MgCl 2 , 50 mM NaCl and 0.2 mM DTT in 50 mM HEPES, pH 8 at 35 °C for 1 h. EDTA was added to 50 mM concentration to quench the reaction. Buffer was exchanged to 20 mM sodium citrate, pH 5.8 using a PD-10 desalting column (GE Healthcare). The charged E2 was immediately loaded onto a HiTrap SP HP column (GE Healthcare). A gradient of 0–1 M NaCl was applied to separate charged E2 from uncharged E2 and ubiquitin. The concentration of conjugate was determined from absorbance at 280 and 504 nm using a NanoDrop ND-1000 spectrophotometer (Thermo Scientific). The charged E2 protein was concentrated, aliquoted and stored at −80 °C until use. A working stock of UbcH5c ∼ BODIPY-FL-Ub (210 nM in 50 mM HEPES, pH 7.2, 50 mM NaCl and 0.01% Triton X-100) was prepared. (Ideally, this working stock should be made daily from material stored at −80 °C. Three or more days after preparation of the working stock, assay quality was observed to deteriorate significantly.) E3 was diluted to 60 μM in 20 mM Tris, pH 7.5, 150 mM NaCl and 1 mM DTT (E3 storage buffer, described above). Lysine was dissolved at the appropriate concentration in 50 mM HEPES, pH 7.2, 50 mM NaCl and 0.0178% Triton X-100. The reaction was conducted in a 21-μl 384-well format (ProxiPlate 384F Plus; PerkinElmer). Lysine stock (9 μl) and E3 (7 μl; 20 μM final) were added to the plate. The reaction was initiated by the addition of 5 μl E2 ∼ BODIPY-FL-Ub (50 nM final) to each well. FP was monitored using a Wallac Victor 3 V reader (PerkinElmer). The maximum polarization (E3–E2 ∼ Ub complex; MAX) was different for each of the six PCGFs and ranged from 188 to 289 mP. The MAX value did not vary significantly for PCGF mutants compared with the WT proteins. The minimum polarization (Ub; MIN) was determined to be 122±4 mP from wells containing 50 nM BODIPY-FL ubiquitin. Observed initial reaction rates in mP min −1 were scaled by dividing by the appropriate MAX–MIN to yield the apparent pseudo first-order rate constant k ′ (in min −1 ). Reactions were conducted for each lysine concentration in duplicate wells; data shown are averages±s.d. for 1–3 independent experiments (that is, 2–6 total replicates). Nucleosome ubiquitination assay Nucleosomes were assembled from the EpiMark Nucleosome Assembly Kit (E5350, NEB) using the dilution assembly protocol. Octamer refers here to histones lacking the DNA component and was produced using the same steps of the dilution assembly protocol as for the nucleosome, but without added DNA. (At lower salt conditions, such as those used in the ubiquitination assay, dissociation of the octamer to H2A–H2B dimers and (H3–H4) 2 tetramers is expected [64] .) E1 (50 nM) (ref. 66 ), 1 μM UbcH5c (Boston Biochem), 300 nM RING1B–PCGF, 20 μM Ub and 150 nM nucleosome or histone octamer (New England Biolabs; NEB) were incubated in 50 mM HEPES pH 7.2, 2.5 mM ATP, 5 mM MgCl 2 , 0.2 mM DTT and 2 mg ml −1 BSA at room temperature for 1 h. Reactions were quenched with LDS sample buffer, and products were resolved on 4–12% NuPAGE Bis-Tris gels run in MES buffer (Life Technologies). Duplicate gels were run and bands were transferred onto nitrocellulose membranes using the iBlot device (Life Technologies). Membranes were blocked with 5% nonfat milk (Bio-Rad) and 1% BSA in 1 × PBS, 0.05% Tween-20 (with rocking at 4 °C, 2 h). All antibody dilutions were made in this solution. Membranes were probed with α-Histone H2A K119ub (Cell Signaling #8240) at 1:1,000 dilution or α-Histone H3 (Cell Signaling #4499) at 1:1,000 dilution (with rocking at 4 °C, overnight). Membranes were rinsed and then washed three times (with rocking at room temperature, 5 min each) with 1 × PBS, 0.05% Tween-20 followed by incubation with α-rabbit-HRP (Cell Signaling #7074) at 1:3,000 dilution (rocking at room temperature, 1 h). Again, membranes were rinsed and then washed three times as above. Bands were visualized using ECL Prime (GE Healthcare). For the inhibition assay with LANA peptides, BSA was omitted from the reaction buffer, and peptides were used at a final concentration of 40 μM (WT LANA peptide sequence: MAPPGMRLRSGRSTGAPLTRGS and LANA LRS mutant peptide sequence: MAPPGMRAAAGRSTGAPLTRGS). For quantitative comparison of E3 variants in the H2A ubiquitination assay, reaction components were as described above with no added BSA, except that the ubiquitin substrate was 10 μM Alexa Fluor 488 ubiquitin (see above) supplemented with 10 μM unlabelled ubiquitin to yield 20 μM final concentration. Products were separated by gel as described above and analysed in parallel by western blot and by imaging of fluorescence on a Typhoon imager (GE Healthcare) with PMT setting 600 and manufacturer settings for Alexa Fluor 488. Fluorescence in gel bands was quantified using the ImageQuant software (GE Healthcare) and corrected for background by subtracting the counts from an area of the same size taken from an adjacent portion of the gel with no bands. A standard curve was generated for each experiment by analysing as above a dilution series of Alexa Fluor 488 ubiquitin together with experimental samples. The comparison of eight PCGF4 and PCGF5 variants was run three times in independent experiments, and data are presented as a mean of background-corrected values at each time point±s.e.m. Generation of UbcH5c(S22R/C85K) ∼ Ub Purified UbcH5c(S22R/C85K) was charged with purified His 6 -Ub in a solution containing 2 μM E1 (ref. 66 ), 200 μM UbcH5c(S22R/C85K), 200 μM ubiquitin, 10 mM ATP, 10 mM MgCl 2 , 0.5 mM TCEP and 50 mM Bis-Tris Propane, pH 9.0 at 37 °C for ∼ 24 h. The product was applied to Ni NTA superflow resin. The resin was washed with 50 mM Tris pH 7.5, 200 mM NaCl, 20 mM imidazole and 1 mM DTT to remove free UbcH5c(S22R/C85K). Free Ub and UbcH5c(S22R/C85K) ∼ Ub were eluted using 50 mM Tris, pH 7.5, 200 mM NaCl, 250 mM imidazole and 1 mM DTT. This was followed by purification over a Superdex 200 column equilibrated in 20 mM Tris pH 7.5, 150 mM NaCl and 1 mM DTT, to separate UbcH5c(S22R/C85K) ∼ Ub from free Ub. Bio-layer interferometry binding measurements Binding measurements were performed by BLI on the OctetRed 384 system (ForteBio). Purified GST–RING1B–PCGF constructs were immobilized onto anti-GST biosensors. Titration series of either UbcH5c(S22R/C85K) or UbcH5c(S22R/C85K) ∼ Ub were used to generate a binding curve. The BLI studies were carried out in 20 mM Tris, pH 7.5, 50 mM NaCl, 1 mM DTT, 0.5 mg ml −1 BSA and 0.01% Tween. To account for any non-specific binding of E2 or charged E2 to sensors, measurements from blank sensors without GST–Ring1b–PCGF were subtracted for each concentration used. Steady-state K D determination was performed using the ForteBio Analysis software (version 7.0) and by non-linear regression using Prism (version 6.0b, GraphPad). Crystallization and structure of RING1B–PCGF5–UbcH5c Purified PCGF5–RING1B was concentrated to 730 μM in a final buffer containing 20 mM Tris 7.5, 100 mM NaCl and 1 mM DTT. Purified UbcH5c was concentrated to 1200 μM in a final buffer containing 50 mM HEPES pH 7.2, 100 mM NaCl and 1 mM DTT. The PCGF5–RING1B complex was mixed with UbcH5c and diluted with 20 mM Tris, pH 7.5, 100 mM NaCl and 1 mM DTT, such that the final concentration of each component was 280 μM. Crystals were obtained by mixing equal volumes of the protein with well solution, using sitting-drop vapour diffusion at 4 °C. The well solution contained 13.5% polyethylene glycol 550 MME, 10 mM TCEP, 0.1 M MES, pH 6.5 and 100 mM KCl. The crystals were flash frozen in the well solution supplemented with 7% glycerol, 7% ethylene glycol and 7% sucrose. Data were collected at ALS 5.0.2. Data were processed with HKL2000 (ref. 66 ). Initial phases were obtained using molecular replacement with the RING1B–UbcH5c portion of the PCGF4–RING1B–UbcH5c complex (chains A and C, PDB code: 3RPG [37] ) as the search model in PHASER [67] . Cycles of model building and refinement were performed in Coot [68] and PHENIX [69] . The structure of PCGF5–RINBG1B–UbcH5c was refined at a resolution of 2.00 Å, with two copies of UbcH5c (chains A and D), RING1B (chains B and E) and PCGF5 (chains C and F). Residues with main chain atoms having poor or missing density were not built. Side chains with poor or missing density were built as alanine. All structure figures were generated with PyMOL (Schrödinger). Refinement statistics are given in Table 2 and were generated with the PHENIX ( Table 1 ) Utility [69] . A representative portion of the electron density map is shown in Supplementary Fig. 12 . Accession codes: Coordinates and structure factors for PCGF5–RING1B–UbcH5c complex have been deposited into the Protein Data Bank under the accession code 4S3O . How to cite this article: Taherbhoy, A. M. et al . BMI1–RING1B is an autoinhibited RING E3 ubiquitin ligase. Nat. Commun. 6:7621 doi: 10.1038/ncomms8621 (2015).